EARLY BUD-BREAK 1 and EARLY BUD-BREAK 3 control resumption of poplar growth after winter dormancy Bud-break is an economically and environmentally important process in trees and shrubs from boreal and temperate latitudes, but its molecular mechanisms are poorly understood. Here, we show that two previously reported transcription factors, EARLY BUD BREAK 1 (EBB1) and SHORT VEGETATIVE PHASE-Like (SVL) directly interact to control bud-break. EBB1 is a positive regulator of bud-break, whereas SVL is a negative regulator of bud-break. EBB1 directly and negatively regulates SVL expression. We further report the identification and characterization of the EBB3 gene. EBB3 is a temperature-responsive, epigenetically-regulated, positive regulator of bud-break that provides a direct link to activation of the cell cycle during bud-break. EBB3 is an AP2/ERF transcription factor that positively and directly regulates CYCLIND3.1 gene. Our results reveal the architecture of a putative regulatory module that links temperature-mediated control of bud-break with activation of cell cycle. The alteration of periods of active growth and dormancy is a widespread adaptive strategy in plants from seasonal climates that enable them to survive unfavorable conditions associated with prolonged periods of low temperature and/or moisture stress. In boreal and temperate woody perennials, winter bud dormancy is developed in the fall and involves, in chronological order: cessation of shoot elongation, the formation of buds (bud-set), and establishment of dormancy. In most woody plants, including Populus , cessation of shoot growth and the induction of dormancy are either induced or accelerated by short days (SDs), and prevented or delayed by long days (LDs) [1] , [2] . The integration of photoperiod detection and growth inhibition involves the convergence of the regulatory activities of the circadian clock machinery (involved in photoperiod sensing) on the FT (FLOWERING LOCUS T) regulatory hub [3] , [4] , [5] , [6] . In poplar, the clock daylength/nightlength sensing components LHY1 (LATE ELONGATED HYPOCOTYL 1), LHY2, GI (GIGANTEA), and CO1/2 (CONSTANS) regulate FT2 (one of two FT paralogs) expression in accordance with the day length [4] , [7] , [8] , [9] . High FT2 expression promotes active growth, while FT2 repression leads to early growth cessation and bud set [6] , [10] . The signaling downstream of FT2 involves Like-APETALA1 (LAP1), which directly and positively regulates AINTEGUMENTA-Like 1 ( AIL1 ) gene [11] , while AIL1 directly regulates D-type cyclins, an important cell cycle progression check point [12] . Thus, growth cessation and bud-set prior to dormancy establishment have co-opted genes and signaling cascades that regulate the photoperiodic floral initiation pathway. Following growth cessation and bud set, continual exposure to SD results in the establishment of a dormant state during which buds are insensitive to growth-promoting signals [13] . It was recently shown that abscisic acid (ABA) plays a major role in the establishment of bud dormancy [14] . Specifically, under SDs, ABA concentration and signaling increase and promote the biosynthesis and deposition of callose at the plasmodesmata (PD) to develop obstructions known as PD sphincters [15] , [16] , [17] , [18] . These symplastic blockages isolate shoot apical meristem (SAM) from growth-promoting signals [14] , [19] . Once dormancy is established, resumption of active growth requires prolonged exposure of the bud to low temperatures [5] , [20] , [21] , [22] . This phase, known as dormancy release, ensures that plants resume growth only after the stable return of favorable growth conditions; in essence, it represents a clock measuring the length of winter [23] . Although both LDs and warm temperatures are required for a return to active growth, the dominant triggering signal is warm temperatures [23] . Therefore, in contrast to growth cessation and dormancy establishment phases, which are photoperiod-regulated processes, dormancy release and reactivation of growth are primarily thermo-regulated processes [24] , [25] . How temperature controls dormancy release and bud-break is poorly understood at the molecular level. The discovery of the Dormancy Associated MADS-box ( DAM ) genes from the evergreen peach mutant has led to speculation that dormancy release and bud-break may share similarities with vernalization [26] . Indeed, DAM genes and MADS-box genes like FLOWERING LOCUS C ( FLC ) are repressed during vernalization, which by low temperatures, and expression changes are correlated with changes in activating/repressive histone modifications [27] , [28] . Furthermore, over-expression of DAM genes causes delayed bud-break similar to how FLC overexpression leads to delayed flowering [29] , [30] , [31] . However, since evergreen mutant does not cease growth in response to SDs, its relevance to dormancy and bud-break remains unclear. Similarly, co-suppression of an apple DAM1 ( MdDAM1 ) led to an inability of the transgenic plants to cease growth and establish dormancy [32] . Recently, another MADS-box gene with homology to SVP in Arabidopsis , named SVP-like ( SVL ), was shown to negatively regulate bud-break [29] . SVL not only regulates bud-break but is also a major hub in the signaling cascade leading to dormancy, downstream of ABA signaling [29] . Expression of SVL is regulated by both SD photoperiod during dormancy initiation and low temperature during dormancy release [29] , [33] . Thus, SVL provides the regulatory link between the photoperiodic and thermo-signaling pathways during the onset of dormancy and its release. Earlier we identified the poplar EARLY BUD-BREAK 1 ( EBB1 ) gene encoding a transcription factor of the AP2/ERF family with high homology to Arabidopsis SAM activity regulator DORNROSCHEN (DRN), as a conserved positive regulator of bud-break [34] , [35] . However, the regulatory context of EBB1 and its link with the SVL pathway remained unclear. As a result, there are significant gaps in our knowledge of how bud-break is regulated. Here, we demonstrate that EBB1 acts as a direct upstream repressor of SVL. Importantly, we identify EBB3, a transcription factor of the AP2/ERF family as a component of the EBB1-SVL bud-break pathway. Our results demonstrate that EBB3 is epigenetically regulated by low temperature and promotes bud-break by positively regulating cell proliferation-related genes. The elucidation of the role of EBB3 thus provides a missing link of low-temperature signals, cell proliferation, and the control of bud-break. Early bud-break 3D mutant discovery A population of activation tagged WT-717 ( Populus tremula X Populus alba ) was screened in a field trial and a mutant with early bud-break was identified (Fig. 1a ). The early bud-break phenotype of the mutant was also validated under controlled growth chamber conditions. Similar to our field observation, mutant plants showed precocious bud-break that was around 6 days earlier as compared to WT-717 (Fig. 1b, d ). Because of the early bud-break phenotype, the mutant was named early bud-break 3 Dominant ( ebb3D ) and the corresponding gene EBB3 ( EARLY BUD-BREAK 3 ). We positioned the tag in the genome sequence on chromosome XII and found two genes (Potri.012G108400 and Potri.012G108500) flanking the insertion within 10Kb up and downstream of the insertion site. Potri.012G108400 was 7.8Kb upstream and Potri.012G108500 2.4Kb downstream of the activation tag insertion (Fig. 1c ). Next, we compared the expression of these two genes in the ebb3D mutant and WT-717 plants. Both genes were upregulated in ebb3D mutants as compared to WT-717 plants (Fig. 1e, f ). Potri.012G108400 encodes a protein similar to ribosomal protein L34e (RPL34e), which is involved in translation and ribosome biogenesis. Potri.012G108500 encodes an AP2/ERF domain-containing transcription factor with similarity to PtERF113 of subfamily B4 (Supplementary Fig. 1 ). Fig. 1: Isolation and molecular analysis of the early bud-break 3D ( ebb3D ) poplar mutant. a ebb3D poplar mutant plants show early bud-break in the field during the start of the second growing season as compared to neighboring WT-717 control trees, arrows point to two ebb3D ramets that show early bud-break compared to the WT-717 plants and other neighboring activation tagging events. b Early bud-break in ebb3D mutant plant as compared to WT-717 under controlled growth chamber conditions (see Methods for more details). c Genome position of the activation tag insertion in the ebb3D mutant, 4X enhancers derived from the CaMV35S promoter. d The average number of days to bud-break in WT-717 and ebb3D mutant plants. e , f Potri.012G108400 and Potri.012G108500 genes are upregulated in the ebb3D mutant. Expression values are the average of three biological replicates ±SEM, normalized to the reference ACT7 gene. At least 10 plants of the ebb3D mutant and WT-717 genotypes were used in the bud-break analysis. Asterisks (*) and (**) indicate significant differences at P < 0.02 and P < 0.002 compared to WT-717 control plants by two-tailed paired t -tests. Source data underlying Fig. 1a–d are provided as a Source Data file. Full size image EBB3 is PtERF113 and its overexpression leads to early bud-break while its suppression causes a delay in bud-break Since both candidate genes were activated in ebb3D mutant we proceeded to pinpoint the causal gene underlying the phenotype by overexpressing them in the parental WT-717 genetic background. A total of 13 Potri.012G108400/RPL34e and 18 Potri.012G108500/PtERF113 overexpressing independent transgenic events were recovered and three lines with high overexpression (Fig. 2b and Supplementary Fig. 2a ) of the two transgenes were tested for the ebb3D phenotype. The overexpression transgenics for Potri.012G108400/RPL34e showed no phenotypic differences compared to WT-717, including the timing of bud-break (Supplementary Fig. 2b ). In contrast, all three Potri.012G108500 /PtERF113-overexpressing lines (EBB3-OE_7, EBB3-OE_9, and EBB3-OE_22) showed significantly early bud-break as compared to WT-717 control plants (Fig. 2a–c ). Therefore, the gene responsible for the ebb3D phenotype is PtERF113, hereafter, referred to as Early Bud-break 3 (EBB3), and transgenic lines overexpressing this gene as EBB3-OE. To further confirm the function of EBB3 in bud-break, we downregulated the expression of EBB3 (EBB3-RNAi). Three independent transgenic lines (EBB3-RNAi) with significantly reduced EBB3 expression were generated. Contrary to EBB3 overexpressers, all three EBB3-RNAi lines (EBB3-RNAi_7, EBB3-RNAi_8, and EBB3-RNAi_10) showed significantly delayed bud-break compared to WT-T89 (Fig. 2d–f ). Taken together, these results show that EBB3 (PtERF113) is a positive regulator of bud-break in poplar. Fig. 2: EBB3 over- and under-expressing lines show early and late bud-break phenotypes respectively. a Early bud-break of a representative over-expressing line compared to WT-717 control plant. b EBB3 relative expression in EBB3-OE lines. c Time to bud-break in WT-717 plants and EBB3-OE lines. d Delayed bud-break in representative EBB3 under-expressing line compared to WT-T89 control plant. e EBB3 relative expression in EBB3-RNAi lines. f Time to bud-break relative to WT-T89 control plants in EBB3-RNAi lines. Expression values are average of three biological replicates ±SEM, normalized to the reference ACT7 for WT-717 and UBQ gene for WT-T89 clones, respectively. Asterisks (*) indicate significant and (**) indicate extremely significant differences compared to WT at P < 0.05 and P < 0.0001, respectively, and determined by two-tailed paired t -tests. Source data underlying Fig. 2a, c, and d are provided as a Source Data file. Full size image EBB3 expression pattern further supports its role in the control of bud-break To better understand the role of EBB3 in the regulation of dormancy we studied its expression pattern during active growth and through a dormancy cycle. EBB3 is highly and primarily expressed in the actively growing shoot apex (Fig. 3a ). We first studied the expression of the gene in wild aspen trees in the field during the activity-dormancy cycle. EBB3 expression was very low during growth cessation and dormancy establishment (Sep–Oct) and highly upregulated during winter/spring months (Nov-March) (Fig. 3b ). This suggests that EBB3 expression may be regulated by low-temperature signals. Consistent with the role of EBB3 as a positive regulator of bud-break, its expression peaks right before or at the time of bud-break in March. Interestingly, EBB3 was precipitously downregulated post-bud-break in April, suggesting a specific functional role in bud-break (Fig. 3b ). To more precisely correlate the expression of EBB3 with different stages of the activity-dormancy cycle in the natural condition, we exposed poplar plants (WT- T89) to a regime of SDs (10WSD: 10 weeks under SD photoperiod) to induce growth cessation and dormancy, followed by exposure to 5 weeks of cold temperatures (4 °C) (5WC) (dormancy release) and 2 weeks of a LD and warm temperature (2WLD) to induce bud-break. EBB3 expression was low in actively growing apices (0 W: time point before inductive treatments) and under SD photoperiod (10WSD) (Fig. 3c ). EBB3 was strongly upregulated after 2 weeks of exposure to low temperature (2WC), remained high after 5 weeks of cold treatment (5WC), and further increased following bud exposure to warm temperature and LD (bud-break) (2WLD) (Fig. 3c ). This indicates that low temperature, which is required for release from dormancy, positively regulates EBB3 expression. Fig. 3: EBB3 is primarily expressed in the shoot apex and differentially regulated during the dormancy cycle and bud-break. a Relative expression of EBB3 in different tissues of WT-717 plants. b Relative expression of EBB3 in vegetative buds of wild-growing aspen ( Populus tremuloides ) trees. c Relative expression of EBB3 in WT-T89 plants under manipulative dormancy treatments in controlled growth chamber conditions. Expression values are the average of three biological replicates ±SEM, normalized to the reference genes ACT7 for WT-717 clones, and UBQ for WT-T89 clones, respectively. 0 W: time point before inductive treatments, 10 WSD: 10 weeks under SD photoperiod, 2WC: 2 weeks under cold, 5WC: 5 weeks under cold, 2WLD: 2 weeks under LD photoperiod and warm temperature. d Average H3K27me3 abundance of three biological replicates in the EBB3 locus, including 2 Kb downstream and upstream regions, before dormancy inductive treatments (0 W) and during dormancy induction, (6WSD, 10WSD) and dormancy release (4WC). H3K27me3 abundance was normalized relative to H3 abundance. Shaded areas indicate ±standard deviation. TSS transcription start site, TTS transcription termination site, cds coding sequence, UTR untranslated region. Source data underlying Fig. 3c are provided as a Source Data file. Full size image Low-temperature induction of EBB3 is epigenetically regulated We then investigated how dormancy release cues such as low temperature could mediate EBB3 expression change. Low temperatures have been found to trigger histone modifications that promote or repress transcription of regulatory genes [36] . It has been previously shown that repressive H3 lysine 27 trimethylation (H3K27me3) histone marks are responsive to cold temperature in peach and pear [27] , [37] . Therefore, we investigated whether EBB3 activation after cold exposure involves changes in H3K27me3. Indeed, the repressive mark H3K27me3 was significantly decreased at the EBB3 locus after exposure to low temperature that promotes dormancy release (Fig. 3d ). The temporal correlation between the decrease in H3K27me3 repressive marks in the EBB3 gene and its upregulation after low-temperature exposure (Fig. 3c ) strongly suggests that H3K27me3 modification plays role in EBB3 regulation during dormancy release. EBB1 directly suppresses SVL expression To better understand how the regulatory roles of EBB1, SVL, and EBB3 (the three known genes that control bud-break) are integrated, we first investigated potential interactions between EBB1 and SVL. We studied the EBB1 and SVL expression during the active growth and dormancy cycle under a controlled environment. EBB1 expression was downregulated under SD photoperiod (10WSD) (Fig. 4a ), strongly upregulated after exposure to low temperature (dormancy release) (5WC), and further increased following exposure of the bud to warm temperatures and LDs (bud-break) (2WLD) (Fig. 4a ). The pattern of SVL expression was opposite to that for EBB1 . SVL expression was relatively high during SDs, repressed by low temperatures and remained low during warm temperatures and LDs (Fig. 4b ). Since the expression profiles of these two genes indicated that they may regulate each other, we studied the expression of SVL in EBB1 over- (EBB1-OE) and under-expressing (EBB1-ami) plants. SVL expression was significantly repressed in EBB1 overexpressers and upregulated in EBB1 downregulated plants (Fig. 4c ). These results indicate that EBB1 may act upstream of SVL to repress its expression. To ascertain if EBB1 directly regulates SVL , we employed EMSAs (Electrophoretic Mobility Shift Essays) to determine if EBB1 binds to the SVL promoter. Since EBB1 is an AP2/ERF transcription factor, binds to a consensus motif (GCCGCCA) known as a GCC-box [38] , we scanned the −2000 bp putative SVL promoter region and found a GCC-box −150 bp from the translation start site (Fig. 4d ). EBB1 bound specifically to the GCC-box (27 bp); no binding occurred with three mutated versions of the GCC-Box (Details in “Methods”, Supplementary Fig. 3 ). These data indicate that EBB1 directly binds to the SVL promoter under in vitro conditions. Further, to confirm in vivo binding of EBB1 to SVL promoter we performed ChIP-qPCR (Chromatin immunoprecipitation-quantitative PCR). Chromatin was isolated from EBB1-GFP DNA transfected poplar protoplasts using an anti-GFP antibody, whereas the IgG antibody was used as control. Consistent with the in vitro EMSA binding assay, the ChIP-qPCR results showed strong binding of EBB1 with the regulatory region of the SVL containing the GCC-box (Fig. 4d ). Thus, the EMSA and ChIP-qPCR results indicate that EBB1 directly binds to the SVL promoter to regulate its expression. Fig. 4: EBB1 directly binds to SVL promoter in vivo in chromatin immunoprecipitation (ChIP) assays to regulate its expression. a EBB1 and b SVL relative expression during dormancy cycle and bud-break under manipulative dormancy treatments in controlled growth chamber conditions; 0 W: time point before inductive treatments, 10WSD: 10 weeks under SD photoperiod, 5WC: 5 weeks under cold, 2WLD: 2 weeks under LD photoperiod and warm temperature. c Relative expression of SVL in EBB1 over-expressing (EBB1-OE) and underexpressed (EBB1-ami) plants. Expression values are the average of three biological replicates ±SEM, the expression values normalized to the reference ACT7 gene. d Enrichment of a DNA fragment in the SVL promoter containing a GCC-box and quantified by ChIP-qPCR. The green box is a schematic representation of the SVL promoter showing the position of the GCC-box (red). Red arrows delineate the position of DNA fragments containing the GCC-box and green arrows demarcate the position of DNA fragments with no GCC-box used as a negative control (NC) in ChIP-qPCR analysis. Chromatin from EBB1-GFP DNA transfected poplar protoplasts was isolated using anti-GFP antibody and IgG used as a control antibody. ChIP-purified DNA was used to perform ChIP-qPCR, expression values are represented as the percentage of input (% of input) DNA. Values are the average of three biological replicates ±SEM. Asterisks (*) and (**) indicate extreme significant differences compared to their respective control at P < 0.003 and P < 0.0005 respectively and determined using two-tailed paired multiple t -tests. Source data underlying Fig. 4d are provided as a Source Data file. Full size image EBB3 is downstream of EBB1 and SVL To determine if EBB3 is part of the EBB1/SVL-mediated regulatory mechanism, we first examined the expression of EBB3 in EBB1 transgenic plants. EBB3 was significantly upregulated in EBB1-OE plants and downregulated in EBB1-ami plants (Fig. 5a ). These data indicate that EBB1, EBB3, and SVL are part of a common regulatory mechanism and that EBB1 acts upstream of SVL and EBB3 to regulate their expression. To determine whether EBB3 acts up- or downstream of SVL, we studied SVL expression in EBB3 overexpressing (EBB3-OE) and downregulated (EBB3-RNAi) transgenic plants. There was no significant change in the expression of SVL in EBB3-OE or EBB3-RNAi plants (Supplementary Fig. 4a, b ). We also performed EMSAs using HA-tagged EBB3 protein and putative binding sites in the SVL promoter, HA-EBB3 does not bind to the SVL promoter (Supplementary Fig. 4c ). Further, we also checked in vivo binding of EBB3 to SVL promoter by ChIP-qPCR assay. Consistent with our in vitro binding assay, no evidence of EBB3 binding to the regulatory region of the SVL was detected (Supplementary Fig. 4d ). These results suggest that EBB3 is downstream of SVL with respect to the regulation of bud-break. To confirm this, we investigated EBB3 expression in SVL transgenics. EBB3 was downregulated in SVL overexpressing (SVL-OE) plants whereas conversely it was upregulated in SVL suppressed (SVL-RNAi) plants (Fig. 5b, c ). These results further confirmed that EBB3 acts downstream of SVL. Fig. 5: EBB1, SVL, and ABA regulate the expression of EBB3 . a Relative expression of EBB3 in EBB1 over-expressing and under-expressing plants. Relative expression of EBB3 in SVL over-expressing ( b ) and under-expressing ( c ) plants. d Relative expression of EBB3 in ABA-treated apices of WT-717 plants. e EBB3 expression in apices of transgenic hybrid aspen with reduced ABA response ( abi1 mutant); 0W: time point before inductive treatments, 10WSD: 10 weeks under SD photoperiod, 5WC: 5 weeks under cold, 2WLD: 2 weeks under LD photoperiod and warm temperature. Expression values are the average of three biological replicates ±SEM, normalized to the reference genes - UBQ for WT-T89 and ACT7 for WT-717 clones respectively. Asterisks (*) indicate significant and (**) indicate extremely significant differences compared to WT at P < 0.04 and P < 0.001 respectively and determined using two-tailed paired multiple t -tests. Full size image Bud-break suppressor ABA negatively regulates EBB3 It was recently shown that ABA is a major regulator of bud dormancy and repressor of bud-break [14] . ABA also positively regulates SVL expression, while SVL in turn positively regulates ABA biosynthesis and signaling-related genes thus forming positive feedforward loop [29] . Therefore, we investigated whether ABA regulates EBB3 expression. Indeed, ABA treatment significantly downregulated EBB3 expression in shoot apices (Fig. 5d ). Furthermore, EBB3 expression in transgenic hybrid aspen with a reduced ABA response ( abi1-1 ) was significantly higher than in WT-T89 plants (Fig. 5e ). Because GA biosynthesis is upregulated in the abi1-1 poplar mutant [14] , we wanted to differentiate whether the elevated EBB3 expression in abi1-1 transgenics is a result of the reduced ABA response or increased GA levels. We, therefore, studied EBB3 expression in GA-treated, WT-717 shoot apices. No significant changes in EBB3 expression were found after GA treatment (Supplementary Fig. 5 ). Thus, these data indicate that EBB3 is a target of ABA signaling downstream of the SVL/ABA feedforward loop during dormancy release and bud-break. Extensive transcriptomic changes are associated with modulation of EBB3 expression during the activity-dormancy cycle To better understand the EBB3 mediated control of bud-break and to identify the downstream target of EBB3 involved in bud-break, we performed transcriptome analysis of EBB3-RNAi transgenics during the activity-dormancy cycle. We focused on apices because of the highest expression of the gene in these tissues. There were 29 differentially expressed genes after dormancy establishment (10WSD), 110 after 5-week cold treatment (5WC), and 1162 at the time of bud-break (2WLD) (Supplementary Data 1 – 7 , Supplementary Table 2 , see also “Methods” for statistical analysis). 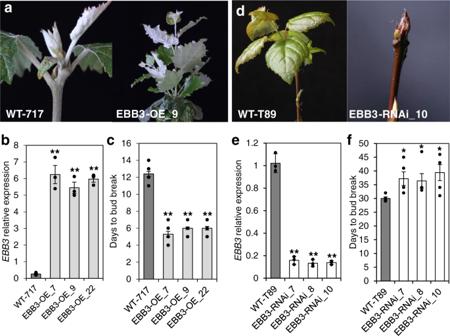Fig. 2: EBB3 over- and under-expressing lines show early and late bud-break phenotypes respectively. aEarly bud-break of a representative over-expressing line compared to WT-717 control plant.bEBB3relative expression in EBB3-OE lines.cTime to bud-break in WT-717 plants and EBB3-OE lines.dDelayed bud-break in representative EBB3 under-expressing line compared to WT-T89 control plant.eEBB3relative expression in EBB3-RNAi lines.fTime to bud-break relative to WT-T89 control plants in EBB3-RNAi lines. Expression values are average of three biological replicates ±SEM, normalized to the referenceACT7for WT-717 andUBQgene for WT-T89 clones, respectively. Asterisks (*) indicate significant and (**) indicate extremely significant differences compared to WT atP< 0.05 andP< 0.0001, respectively, and determined by two-tailed pairedt-tests. Source data underlying Fig.2a, c, and dare provided as a Source Data file. The number of differentially expressed genes in the different dormancy stages corresponds well with the native EBB3 expression level during dormancy release and bud-break. EBB3 directly regulates CYCD3.1 gene expression The CYCD3.1 (Potra002502g18897) gene was the only gene among all differentially regulated genes, that was statistically significantly ( P < 0.05) downregulated in the EBB3-RNAi plants at all time points studied using RNA-seq (Fig. 6a , Supplementary Data 4 – 7 ). We, therefore, studied the expression of the CYCD3.1 gene in EBB3-OE plants using qRT-PCR and found that in contrast to EBB3-RNAi plants where the gene was significantly downregulated, CYCD3.1 was significantly upregulated in EBB3-OE plants (Fig. 6b ). These data further suggested that CYCD3.1 is downstream of EBB3. EBB3 is an AP2/ERF transcription factor that binds to a consensus GCC-box [38] , and we identified a GCC-box-like (GCCGGGCCA) motif in the promoter region of CYCD3.1 . To confirm that CYCD3.1 is a direct target of EBB3, we performed EMSA using 6xHIS-tagged EBB3-purified protein and the 27 bp GCC-box. The EBB3 protein specifically bound the GCC-box fragment of the CYCD3.1 promoter, whereas no binding was observed with the mutated version of the GCC-Box (TCCTTTCCA) (Supplementary Fig. 6 ). Further, we checked in planta EBB3 binding to the GCC-box of CYCD3.1 promoter using ChIP-qPCR assays in poplar protoplasts. EBB3 showed clear binding to the part of CYCD3.1 promoter containing the GCC-box (Fig. 6c ). These results show that EBB3 positively and directly regulates CYCD3.1 expression during dormancy release and bud-break. Fig. 6: EBB3 binds directly to the CYCD3.1 promoter in vivo in chromatin immunoprecipitation assays to regulate its expression. a Number of common and unique downregulated genes in EBB3 RNAi under-expressing plants in different dormancy stages. The Cyclin D3.1 ( CYCD3.1 ) is the only downregulated gene in all dormancy stages. See Supplementary Data 4 – 7 for more details. b Relative expression of CYCD3.1 in EBB3-OE and WT-717 plants; 0W: time point before inductive treatments, 10WSD: 10 weeks under SD photoperiod, 5WC: 5 weeks under cold, 2WLD: 2 weeks under LD photoperiod and warm temperature, expression values are normalized to the ACT7 gene. Expression values are the average of three biological replicates ±SEM. c Enrichment of a DNA fragment in the CYCD3.1 promoter containing a GCC-box and quantified by ChIP-qPCR. The green box is a schematic representation of the CYCD3.1 promoter showing the position of the GCC-box (red). Red arrows delineate the position of DNA fragments containing the GCC-box and green arrows demarcate the position of DNA fragments with no GCC-box used as a negative control (NC) in ChIP-qPCR analysis. Chromatin from EBB3-GFP DNA transfected poplar protoplasts was isolated using anti-GFP antibody and IgG used as a control antibody. ChIP-purified DNA was used to perform ChIP-qPCR, expression values are represented as percentage input (% input) DNA. Values are the average of three biological replicates ±SEM. Asterisks (*) and (**) indicate significant differences compared to their respective control at P < 0.05 and P < 0.004 respectively and determined using two-tailed paired multiple t -tests. Source data underlying Fig. 6a and c are provided as a Source Data file. Full size image We report the identification of a putative regulatory pathway comprised of three transcription factors (EBB1, SVL, and EBB3) that mediate bud-break in poplar (Fig. 7 ). Our gene expression data, in vivo/in vitro binding assays, and analysis of gain- and loss-of-function transgenics indicate that EBB1 acts at the top of the pathway and represses the expression of its direct downstream target SVL . Our data clearly show that hierarchically, SVL/ABA reinforcing loop acts upstream of EBB3 and negatively regulates its expression. Downstream, EBB3 directly and positively regulate CYCLIND3.1 ( CYCD3.1 ), a key promoter of the G1/S progression of the cell cycle whose expression correlates with bud reactivation of growth at bud-break [20] , [39] . The identification of these regulatory interactions would benefit further from in planta analysis of their spatiotemporal specificity during dormancy-activity cycle. Furthermore, genetic evidence derived from double and triple mutants is needed to confirm the functionality and hierarchy of the proposed model. Fig. 7: Hypothetical model of the roles EBB1, SVL and EBB3 play in control of bud-break in poplar. EBB1 is positively regulated by low temperature, leading to suppression of SVL expression. Declining SVL expression breaks the SVL/ABA feedforward loop. SVL/ABA repression leads to the upregulation of EBB3 and consequently to activation of CYCD3.1 , cell proliferation, and bud-break. Green arrows indicate positive regulation while red bars indicate negative regulation. Dash arrows indicate indirect regulation. See the text for additional description. Full size image While EBB1 and SVL were previously discovered as regulators of bud-break [29] , [34] , here we elucidated the interaction between these two components of the bud-break pathway by showing that EBB1 directly and negatively regulates SVL expression. This regulation is likely most relevant at the activity-dormancy transitions as suggested by the dramatic and opposing changes in the expression of these two genes that occur at these transition periods. EBB1 is downregulated, while SVL is upregulated during dormancy induction and establishment (Fig. 4 ). Thus, SVL upregulation during dormancy is, at least in part, due to de-repression brought about by declining levels of EBB1 . Previous work has shown that SVL is also highly ABA responsive and that ABA does increase during dormancy establishment [14] , [16] , [18] , [29] . Thus, SVL upregulation is a result of the combined and opposing regulatory activities of EBB1 and ABA. This situation is gradually reversed during dormancy release and bud-break. EBB1 is upregulated while SVL is downregulated, suggesting that EBB1 after cold treatment re-establishes SVL repression, and this at least in part restores shoot apex competence for growth (Fig. 4 ). SVL and ABA form a feedforward loop; SVL upregulates expression of NCED3 (a critical ABA biosynthetic gene), while ABA upregulates expression of SVL [29] . Rising EBB1 levels during dormancy release likely break this feedforward loop by downregulating the expression of SVL and consequently ABA levels. Thus, EBB1 not only affects SVL expression but also likely indirectly plays a part in reducing the concentration of ABA during chilling to release apices from dormancy. We also report the identification and characterization of EBB3, a component of the EBB1-SVL-mediated regulatory mechanism, that controls bud-break. We present several lines of evidence that clearly implicate EBB3 in the regulation of bud-break. First, transgenic up and downregulation of the gene leads to accelerated and delayed bud-break of the transgenic plants compared to WT controls (Fig. 2 ). EBB3 expression highly correlates with dormancy release and bud-break. EBB3 is almost undetectable during dormancy establishment and significantly increases with the progression of the cold treatment peaking right around the bud-break time. EBB3 encodes a transcription factor of the AP2/ERF family with highest homology to AtERF114, known as ERF BUD ENHANCER (EBE) [40] . In Arabidopsis , EBE is a positive regulator of axillary bud outgrowth [40] . Apical dominance plays a central role in axillary bud dormancy in Arabidopsis [41] . In contrast, winter bud dormancy is imposed by environmental cues and requires resetting through a cold treatment [23] . Thus, it is likely that dormancy regulation in the axillary and apical bud may be different, particularly upstream of EBB3/EBE. Nevertheless, the downstream processes controlled by the two genes appear to share significant similarities. For example, in Arabidopsis , one of the most prominent transcriptomic changes in response to inducible EBE upregulation involves cell cycle genes, including CYCDs [40] . Thus, both EBE and EBB3 appear to activate cell cycle. In Arabidopsis , the genes differentially regulated by EBE have an overrepresentation of TCP18/BRC1 binding sites [40] . It was previously found that in poplar, SVL positively regulates TCP18/BRC1 during dormancy. In Arabidopsis , Class II TCPs, to which BRC1 belongs, repress organ growth by inhibiting cell proliferation at the G1-to-S transition [42] , [43] . Here we find that SVL negatively regulates EBB3 . Thus, the increasing and decreasing abundance of SVL during dormancy can act in balancing cell proliferation and bud-break competence by regulating TCP18/BRC1 and EBB3 . Higher TCP18/BRC1 levels may inhibit cell proliferation and negatively regulate bud-break [44] , while high EBB3 levels post cold treatment would activate cell cycle and bud-break. Although temperature cues have been known to regulate dormancy release and subsequent bud-break, how temperature controls these transitions has not been entirely clear. Interestingly, epigenetic changes at EBB3 locus correlate with gene expression and exposure to dormancy releasing low-temperature signal. Our data show that following exposure to low temperature, there is a reduction in the repressive H3 lysine 27 trimethylation (H3K27me3) marks across the whole sequence of the EBB3 gene with simultaneous upregulation of EBB3 (Fig. 3d ). Low temperatures have been found to trigger histone modification which promotes or represses transcription during vernalization and bud dormancy release [36] . For example, H3 lysine 27 trimethylation (H3K27me3) histone marks in pear EBB1 and peach DAM genes are responsive to cold temperature [27] , [37] . This correlation between repressive marks and expression is not perfect and indicates that EBB3 is under complex regulatory mechanism including but not limited to epigenetic modifications. For example, transcription activators may upregulate the gene prior and at bud-break but repressors downregulate the gene past bud-break. Thus, the summary of all data strongly implicate EBB3 in the regulation of bud-break in poplar and this may involve at least in part low temperature-responsive changes in EBB3 expression via epigenetic changes. The importance of epigenetic changes in the regulation of low-temperature response and bud-break was also recently demonstrated by the role of a poplar DEMETER-LIKE 10 (DML), a DNA demethylase, plays in the regulation of bud-break [45] . To find potential commonalities in the mechanisms governed by EBB3 and DML during bud-break, we compared the differentially expressed genes (DEGs) in EBB3 and DML knocked-down transgenics. A total of 106 common genes were discovered (Supplementary Data 8 ). Analysis of the putative function of the common genes shows gene ontology (GO) terms enrichment (FDR < 0.05) of genes involved in various metabolic processes (Supplementary Data 9 ) but does not show enrichment of genes involved in regulation of cell cycle or growth. This is not surprising as the two genes have very different regulatory activities and likely target different processes during bud-break. Although here we describe regulatory interactions involving mainly transcription control, it is clear that there are multiple diverse regulatory layers that differentially act on the different components of the cascade. For example, low temperatures affect the expression of all three genes (EBB1, SVL, and EBB3). In Arabidopsis , low-temperature signaling is associated with changes in repressive and activation histone marks at MADS-box genes like SVP , which induces flowering after cold [46] , [47] . In sharp contrast, the poplar SVP-like (SVL), a MADS-box gene that regulates bud-break, is not regulated by histone marks [29] , while both EBB1 and EBB3 seem to be regulated by histone modifications [48] (Fig. 3d ). Thus, although the three genes appear to be in a common regulatory module, their larger regulatory context is different. SVL is subject to hormonal, while EBB1 and EBB3 to chromatin and hormonal regulation. The discovery of the three genes and their interactions opens the door for a more comprehensive characterization of the genetic mechanisms regulating bud-break and enables approaches to modify dormancy-associated traits in shrubs and forest and fruit trees from temperate and boreal latitudes more rapidly and strongly. Such breeding and biotechnological approaches may become increasingly important in the face of rapid climate change, whose pace is likely to exceed the capacity of the forests to adapt through natural selection alone [49] . Poor synchronization of bud phenology with local climates can lead to significant damage from early and late frosts, poor crop yields, and the outbreak of pest and disease problems. A better understanding of the molecular mechanisms of the processes involved will allow for knowledge-based approaches to mitigate existing challenges. Mutant ebb3D discovery A poplar activation tagging population was generated and screened [34] , [50] . The EARLY BUD-BREAK3D ( ebb3D ) mutant was discovered in a field trial with 2-year-old plants in which all 4 ramets (arranged in 2 randomly distributed blocks with 2 ramets each) of the line flushed earlier than wild type. The early bud-break phenotype of the ebb3D mutant line was validated in a controlled growth chamber experiment, as described below. Molecular characterization of the mutant The sequence flanking the insertion of the activation tag was recovered using TAIL-PCR [34] , [50] . The recovered sequence was positioned in the poplar genome by BLAST searches and proximal genes to the insertion site were studied for activation by comparing their expression in the ebb3D mutant and wild type plants (see below for details of the expression analysis). Plant material, growth conditions, and phenotypic measurements Hybrid clones 717-IB4 ( Populus tremula x alba; wildtype/WT-717) and T89 ( Populus tremula x tremuloides; wildtype/WT-T89) were used in the experiments. The EBB1-OE line generated in the WT-717 background, and the SVL-OE and SVL-RNAi lines were generated in the WT-T89 background [29] , [34] . Plants were first cultivated in vitro in half-strength MS medium (Duchefa) under sterile conditions for 5 weeks and then transferred to small pots with soil for 2 weeks for acclimation to greenhouse conditions. Plants were then transferred to 2 L pots and grown for 4 weeks in the greenhouse (16-h light, 20 °C) before the manipulative dormancy experiments. 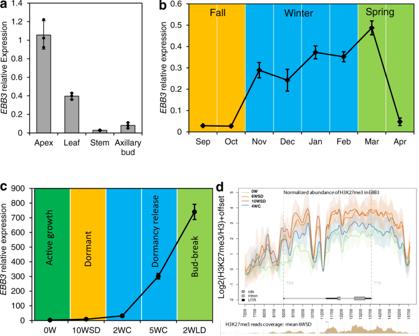Fig. 3:EBB3is primarily expressed in the shoot apex and differentially regulated during the dormancy cycle and bud-break. aRelative expression ofEBB3in different tissues of WT-717 plants.bRelative expression ofEBB3in vegetative buds of wild-growing aspen (Populus tremuloides) trees.cRelative expression ofEBB3in WT-T89 plants under manipulative dormancy treatments in controlled growth chamber conditions. Expression values are the average of three biological replicates ±SEM, normalized to the reference genesACT7for WT-717 clones, andUBQfor WT-T89 clones, respectively. 0 W: time point before inductive treatments, 10 WSD: 10 weeks under SD photoperiod, 2WC: 2 weeks under cold, 5WC: 5 weeks under cold, 2WLD: 2 weeks under LD photoperiod and warm temperature.dAverage H3K27me3 abundance of three biological replicates in theEBB3locus, including 2 Kb downstream and upstream regions, before dormancy inductive treatments (0 W) and during dormancy induction, (6WSD, 10WSD) and dormancy release (4WC). H3K27me3 abundance was normalized relative to H3 abundance. Shaded areas indicate ±standard deviation. TSS transcription start site, TTS transcription termination site, cds coding sequence, UTR untranslated region. Source data underlying Fig.3care provided as a Source Data file. For growth cessation and dormancy induction, plants were transferred from the greenhouse to growth chambers and grown for 10 weeks under short-day (SD) photoperiod (8-hour light, 20 °C /16-h dark, 18 °C). Height, numbers of leaves formed after initiation of SD treatment and bud-set at the apex were recorded weekly [34] Dormant plants were then placed in a cold room at 4 °C for 5 weeks to meet the chilling requirement. To induce bud-break, plants were transferred to warm temperature and LD photoperiod (16-h light, 20 °C/8 h dark, 18 °C). Bud-break of the apical bud was monitored and scored daily [34] . Generation of plasmid constructs and transformation EBB3 full-length CDS was amplified using ebbD3attB1 forward 5′-GGGGACAAGTTTGTAC AAAAAAGCAGGCTATGGATGTGATGGTTTCAGCTC-3′ and ebb3DattB2 reverse 5′-GGG GACCACTTTGTACAAGAAAGCTGGGTTCAAAGCCCCTCGTCTTTGTAT-3′ primers and similarly, RPL34e using RPL34eattB1 forward 5′-GGGGACAAGTTTGTACAAAAAAGCAG GCTATGGTGCAGCGTCTGACTTAC-3′ and RPL34eattB2 reverse 5′-GGGGACCACTTTGTACAAGAAAGCTGGGTTCATTTTGAGGCCTGTTTTTCCT-3′ primers containing B1 and B2 recombination site sequences, respectively. The amplified fragments were first cloned into pDONR221 and then into destination vector pK2GW7 (CaMV 35S promoter) using Gateway BP and LR recombination reactions respectively (Invitrogen). The constructs were sequence-verified and transformed into Agrobacterium strain C58 using the freeze-thaw method [51] . To generate the EBB3-RNAi construct, a 200 bp fragment was amplified using full-length the EBB3 cDNA as a template and the following primers (Forward 5′-CACCTCTGGC GGGACCGAAT-3′ and Reverse 5′-GCAGGCGGCATGACATGGCT-3′). The amplified fragment was cloned into pENTR/D-TOPO (Invitrogen), sequence verified, and then transferred into the plant transformation vectors (CaMV 35S promoter) to generate the EBB3-pK7GWIWG2 (I) construct, which was then transformed into Agrobacterium strain GV3101pmp90RK [52] . The EBB3-RNAi construct was transformed into WT-T89 and whereas EBB3-pK7GWIWG2 (I) construct was into WT-717 plants [53] , [54] . 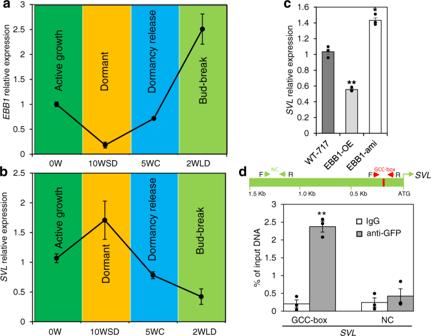Fig. 4: EBB1 directly binds toSVLpromoter in vivo in chromatin immunoprecipitation (ChIP) assays to regulate its expression. aEBB1andbSVLrelative expression during dormancy cycle and bud-break under manipulative dormancy treatments in controlled growth chamber conditions; 0 W: time point before inductive treatments, 10WSD: 10 weeks under SD photoperiod, 5WC: 5 weeks under cold, 2WLD: 2 weeks under LD photoperiod and warm temperature.cRelative expression ofSVLin EBB1 over-expressing (EBB1-OE) and underexpressed (EBB1-ami) plants. Expression values are the average of three biological replicates ±SEM, the expression values normalized to the referenceACT7gene.dEnrichment of a DNA fragment in theSVLpromoter containing a GCC-box and quantified by ChIP-qPCR. The green box is a schematic representation of theSVLpromoter showing the position of the GCC-box (red). Red arrows delineate the position of DNA fragments containing the GCC-box and green arrows demarcate the position of DNA fragments with no GCC-box used as a negative control (NC) in ChIP-qPCR analysis. Chromatin from EBB1-GFP DNA transfected poplar protoplasts was isolated using anti-GFP antibody and IgG used as a control antibody. ChIP-purified DNA was used to perform ChIP-qPCR, expression values are represented as the percentage of input (% of input) DNA. Values are the average of three biological replicates ±SEM. Asterisks (*) and (**) indicate extreme significant differences compared to their respective control atP< 0.003 andP< 0.0005 respectively and determined using two-tailed paired multiplet-tests. Source data underlying Fig.4dare provided as a Source Data file. For expression analysis during the dormancy cycle, we collected vegetative apical buds from small branches of three individual wild aspen ( Populus tremuloides , ~20-years old) trees for each month of the dormancy period (September to April). Whole buds were immediately frozen in liquid nitrogen. For tissue-specific expression analysis, different tissue samples were collected from greenhouse grown four months old WT-717 plants and stored at −80 °C until processed. In control condition experiments, shoot apices for gene expression analyses were collected at the same time of the day (i.e., 15:00 h), after 0, 10WSD, 2WC, 5WC, and 2WLD frozen in liquid nitrogen, and stored at −80 °C. To generate GFP-tagged version of EBB1 and EBB3 DNA, we amplified EBB1 and EBB3 CDSs using gene specific primers (EBB1_B1F: 5′-GGGGACAAGTTTGTACAAAAAAGCAGGCTATGGAAGAAGCGCTTAGAAG-3′, EBB1_B2R: 5’-GGGGACCACTTTGTACAAGAAAGCTGGGTTAAAGCTGGCAGCAAAGGCACT-3′ and EBB3_B1F: 5′-GGGGACAAGTTTGTACAAAAAAGCAGGCTATGGATGTGATGGTTTCAGC-3′, EBB3_B2R: 5′-GGGGACCACTTTGTACAAGAAAGCTGGGTTAAGCCCCTCGTCTTTGTATT-3′) containing B1 and B2 recombination site sequences, respectively. The amplified fragments were cloned into destination vector pMDC83 (CaMV 35S promoter) using Gateway LR recombination reaction (Invitrogen). The sequence-verified plasmids were then used for the poplar protoplast transfection assays. Hormone treatments For the ABA treatment, apices were cut and placed in MS solution with or without 50 µM ABA for 2 h and were then sampled for RNA extraction and expression analysis. For gibberellin (GA) treatments, 3 mM GA 3 solution was applied directly to the shoot apex and sampled after 24 h for expression analysis [55] . RNA isolation and quantitative real-time PCR analysis Total RNA was extracted using an RNeasy® Plant Mini Kit (Qiagen), or an Aurum Total RNA kit (Bio-Rad), or an RNeasy® Plus Universal Kit (Qiagen). Total RNA (10 µg) was treated with RNase-Free DNase (Qiagen) and cleaned using an RNeasy® Mini Kit (Qiagen). 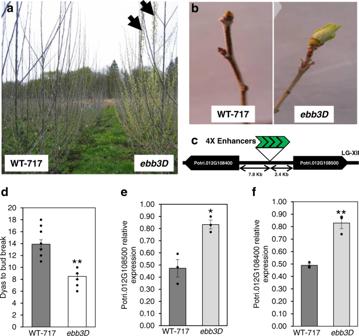One µg of the RNA was used to generate cDNA using an iScript cDNA synthesis kit (Bio-Rad) or SuperScriptII (Invitrogen, Life Technologies). ACT7 (WT-717 background) and ubiquitin ( UBQ ) (WT-T89 background) genes were selected and validated using geNorm Software [56] as a reference gene. qRT-PCR analyses were carried out with StepOnePlus Real-Time PCR System (Applied Biosystems, Life Technologies) and Light Cycler 480 II (Roche) using Maxima SYBR Green qPCR Master Mix (Thermo Fisher Scientific Co.) and relative expression values were calculated using the ∆-Ct-method [12] . Fig. 1: Isolation and molecular analysis of theearly bud-break 3D(ebb3D) poplar mutant. aebb3Dpoplar mutant plants show early bud-break in the field during the start of the second growing season as compared to neighboring WT-717 control trees, arrows point to twoebb3Dramets that show early bud-break compared to the WT-717 plants and other neighboring activation tagging events.bEarly bud-break inebb3Dmutant plant as compared to WT-717 under controlled growth chamber conditions (see Methods for more details).cGenome position of the activation tag insertion in theebb3Dmutant, 4X enhancers derived from the CaMV35S promoter.dThe average number of days to bud-break in WT-717 andebb3Dmutant plants.e,fPotri.012G108400 and Potri.012G108500 genes are upregulated in theebb3Dmutant. Expression values are the average of three biological replicates ±SEM, normalized to the referenceACT7gene. At least 10 plants of theebb3Dmutant and WT-717 genotypes were used in the bud-break analysis. Asterisks (*) and (**) indicate significant differences atP< 0.02 andP< 0.002 compared to WT-717 control plants by two-tailed pairedt-tests. Source data underlying Fig.1a–dare provided as a Source Data file. A complete list of the primers used for RT-PCR is presented in Supplementary Table 1 . Populus protoplast isolation and DNA transfection WT-717 poplar plants were grown in low light (60 µmol/m 2 ) for 6–8 weeks and around 20 fully expanded leaves (1 g) were used to isolate protoplast [57] , [58] . Briefly, fully expanded leaves were cut into 0.5–1 mm fine strips and digested in 40 mL of enzyme solution (cellulase R10 3%, macerozyme R10 0.8%) in dark for 4–5 h without shaking and later 30 min shaking at 50 rpm to release the protoplasts. The protoplasts were harvested and diluted to a concentration of 4 × 10 7 protoplast mL −1 . The plasmids used in transfections were isolated using Qiagen Plasmid Midi Kit (Qiagen Inc.), and 40 µg of EBB1-GFP (EBB1-pMDC83) and 50 µg of EBB3-GFP (EBB3-pMDC83) plasmid DNA added to 500 µL (2 × 10 7 protoplasts) of protoplast for each transfection assays. [58] After transfection, protoplasts were incubated in dark for 20 h and then 4 h on ice. Successful expression of the GFP-tagged proteins was monitored by examining GFP fluorescence of the transfected poplar protoplasts using Olympus SZX16 (Center Valley, PA, USA) (Supplementary Fig. 7 ). Chromatin immunoprecipitation assays After transfection and successful validation of GFP fluorescence, protoplasts were harvested by centrifugation at 200 × g , and the pellet washed with ice-cold 1× PBS. Formaldehyde (1% final concentration) was used to crosslink the protein to DNA, and 125 mM glycine was used to stop the reaction. The crosslinked protoplasts were used to isolate the chromatin using EpiQuick ChIP Kit (EPIGENTEK, P-2002). Anti-GFP (Abcam, Cat No. ab290) and IgG (negative control, provided with kit) antibodies were used for chromatin immunoprecipitation. The enrichment of bound target sequences was quantified by qRT-PCR using the DNA recovered from anti-GFP and IgG ChIPs and normalized against 5% input DNA. All ChIP experiments were carried out in three biological replicates. Generation of labeled SVL promoter fragments and EMSAs with EBB1 and EBB3 proteins Sequence analysis of the SVL promoter showed the presence of an ERF binding site (GCC-box, GCCGCCA) ~150 bp upstream (−150 bp) of the translation start site. Two sets of primers that can amplify 150 bp fragments, one with the binding site and the other without the binding site were amplified by using biotin-labeled primers (see Supplementary Table 1 ) and P. trichocarpa genomic DNA. The fragments were purified using an E.Z.N.A. Gel Purification Kit (Omega Bio-tek) prior to use in gel-shift assays. EMSAs were performed using biotin-labeled promoter fragments and cell extracts from Arabidopsis protoplasts expressing HA-EBB1/HA-EBB3 or control extracts from non-transformed protoplasts [11] . After confirming that HA-EBB1/HA-EBB3 bound to the SVL promoter fragment, smaller, biotin-labeled F1 fragments (27 bp) containing the GCC-box (GCCGCC) or a mutated version of the GCC-box were synthesized. For the EMSA reaction, 10 μL protoplast cell extract was mixed with 0.5 μL biotin-labeled DNA (10 fmol/mL), 0.4 μL nonspecific competitor (poly [dI:dC], 1 mg/mL), and 0.5 μL BSA (20 mg/mL) in EMSA buffer. To determine binding specificity, mutated GCC-box fragments were also used. The mixtures were incubated on ice for 10 min followed by 30 min at room temperature to allow binding. The samples were then separated on a non-denaturing polyacrylamide gel (5%) prepared with 0.5XTBE and transferred to a Hybond N + membrane (GE Healthcare). Finally, a Light Shift Chemiluminescent EMSA kit (Pierce) was used for cross-linking and detection. Generation of CYCD3.1 GCC-box probe and EMSAs with EBB3 protein The CDS of PtaEBB3 was amplified using forward 5′-AAAAGAATTCATGGATGT GATGGTTT-3′ and reverse 5′-AAAAGCGGCCGCAAGCCCCTCGTCTTTG-3′ primers and cloned into the pET32a(+) vector at the EcoRI / NotI sites. The construct was sequenced validated and transformed into One Shot™ BL21(DE3) E. coli cells (Invitrogen). Colonies growing on selection media were validated using PCR and restriction digests. 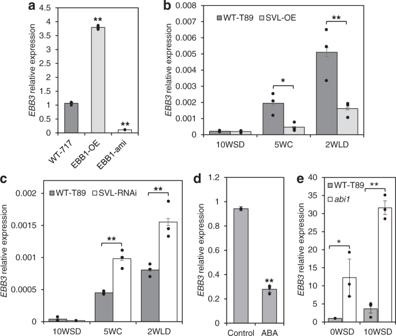Fig. 5: EBB1, SVL, and ABA regulate the expression ofEBB3. aRelative expression ofEBB3in EBB1 over-expressing and under-expressing plants. Relative expression ofEBB3in SVL over-expressing (b) and under-expressing (c) plants.dRelative expression ofEBB3in ABA-treated apices of WT-717 plants.eEBB3expression in apices of transgenic hybrid aspen with reduced ABA response (abi1mutant); 0W: time point before inductive treatments, 10WSD: 10 weeks under SD photoperiod, 5WC: 5 weeks under cold, 2WLD: 2 weeks under LD photoperiod and warm temperature. Expression values are the average of three biological replicates ±SEM, normalized to the reference genes -UBQfor WT-T89 andACT7for WT-717 clones respectively. Asterisks (*) indicate significant and (**) indicate extremely significant differences compared to WT atP< 0.04 andP< 0.001 respectively and determined using two-tailed paired multiplet-tests. Successfully validated colonies were used to inoculate 50 mL LB medium grown for 2 h at 37 °C to obtain an OD 600 between 0.6 and 0.8 and then induced for 20 h with 0.1 mM IPTG (Isopropyl β- d- thiogalactoside) at 16 °C. The PtaEBB3-His protein was purified on Ni 2+ ‐NTA agarose resin (Qiagen) following the manufacturer’s protocol. Forward and reverse primers containing the ERF binding site (GCC-box, GCCGGGCCA) were synthesized (Eurofins Genomics). The double‐stranded probe was prepared by annealing the forward and reverse primers. The EMSA assay was carried out using the Electrophoretic Mobility-Shift Assay (EMSA) Kit, with SYBR™ Green and SYPRO™ Ruby EMSA stains (Invitrogen), according to the product instructions. Protein-DNA complex samples were loaded onto a 4–20% gradient polyacrylamide native gel (Bio-Rad) and run at 100 V for 1 h. The amount of DNA and protein used in the various experiments are indicated in Fig. 6 . The nucleic acid in the gel was stained using SYBR® Green and visualized using a Gel Doc-It (UVP). The primers used for the EMSA analysis are listed in Supplementary Table 1 . ChIP-seq experiment To perform ChIP-seq experiment, apical buds from WT plants of three biological replicates were collected from before dormancy inductive treatments (0 W), after 6 and 10 weeks under SD conditions (6WSD and 10WSD), and again after an additional 4 weeks of cold treatment (4WC). Anti-trimethyl-Histone H3 (LysK27) (Millipore, Cat No. #07-449) and anti-Histone H3 (Abcam, Cat No. ab1791) antibodies were used for chromatin immunoprecipitation. Paired-end (PE) sequencing was done by BGI-Tech. Sequencing reads were processed following the guidelines described at http://www.epigenesys.eu/en/protocols/bio-informatics/1283-guidelines-for-rna-seq-data-analysis . Reads quality was assessed using FastQC ( http://www.bioinformatics.babraham.ac.uk/projects/fastqc/ ), v0.11.4. Ribosomal RNA (rRNA) reads were quantified and filtered using SortMeRNA [59] . Reads were filtered to remove adapters and trimmed for quality using Trimmomatic and then mapped to the Populus genome using STAR [60] , [61] . Then reads were remapped using BWA-MEM [62] and peaks were called genome-wide using MACS2 [63] with the non-default parameters [29] , on sequencing libraries down-sampled to 10 million PE reads. The depth of this down-sampled library was estimated by an ad hoc saturation/rarefaction analysis based on the number of peaks identified by MACS2 in varying subsets of the original dataset. These downstream analyses were solely used to estimate the fraction of the genome mapped under the different growing conditions. The data were normalized using ratios obtained for the analysis of the EBB3 locus histone methylation status. Reads mapped to the sequence of the EBB3 gene including 2 kb upstream and downstream region were extracted from the alignment. Coverage was calculated in the above region, transformed to log2, and corrected for the abundance differences between samples (i.e., the fraction of the genome mapped under the different growing conditions in the 10 M PE read subset; the latter selection addressing any library size factor scaling otherwise required). Finally, the H3K27me3 abundance was normalized by H3 abundance, the mean of three biological replicates was calculated and curves were fitted to the data by local polynomial regression. R [64] and Bioconductor [65] were used to compare differences in histone methylation between the time points. RNA sequencing and differential expression analyses Illumina HiSeq 2500 was used to perform RNA-seq for 125 cycles in paired-end mode at BGI (Beijing, China) using RNA isolated from apices of wild type and EBB3-RNAi at 10 weeks SD, 2 W, and 5 W cold and 2 W LDs. Briefly, the quality of the raw sequence data was assessed using FastQC ( http://www.bioinformatics.babraham.ac.uk/projects/fastqc/ ). Residual ribosomal RNA (rRNA) contamination was assessed and filtered using SortMeRNA [59] (settings --log --paired_in --fastx--sam --num_alignments 1) using the rRNA sequences provided with SortMeRNA (rfam-5s-database-id98.fasta, rfam-5.8s-database-id98.fasta, silva-arc-16s-database-id95.fasta, silva-bac-16s-database-id85.fasta, silva-euk-18s-database-id95.fasta, silva-arc-23s-database-id98.fasta, silva-bac-23s-database-id98.fasta and silva-euk-28s-database-id98.fasta). 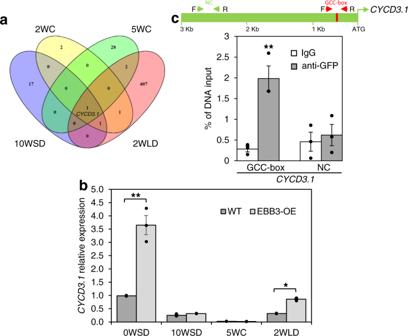Fig. 6: EBB3 binds directly to theCYCD3.1promoter in vivo in chromatin immunoprecipitation assays to regulate its expression. aNumber of common and unique downregulated genes in EBB3 RNAi under-expressing plants in different dormancy stages. TheCyclin D3.1(CYCD3.1) is the only downregulated gene in all dormancy stages. See Supplementary Data4–7for more details.bRelative expression ofCYCD3.1in EBB3-OE and WT-717 plants; 0W: time point before inductive treatments, 10WSD: 10 weeks under SD photoperiod, 5WC: 5 weeks under cold, 2WLD: 2 weeks under LD photoperiod and warm temperature, expression values are normalized to theACT7gene. Expression values are the average of three biological replicates ±SEM.cEnrichment of a DNA fragment in theCYCD3.1promoter containing a GCC-box and quantified by ChIP-qPCR. The green box is a schematic representation of theCYCD3.1promoter showing the position of the GCC-box (red). Red arrows delineate the position of DNA fragments containing the GCC-box and green arrows demarcate the position of DNA fragments with no GCC-box used as a negative control (NC) in ChIP-qPCR analysis. Chromatin from EBB3-GFP DNA transfected poplar protoplasts was isolated using anti-GFP antibody and IgG used as a control antibody. ChIP-purified DNA was used to perform ChIP-qPCR, expression values are represented as percentage input (% input) DNA. Values are the average of three biological replicates ±SEM. Asterisks (*) and (**) indicate significant differences compared to their respective control atP< 0.05 andP< 0.004 respectively and determined using two-tailed paired multiplet-tests. Source data underlying Fig.6a and care provided as a Source Data file. 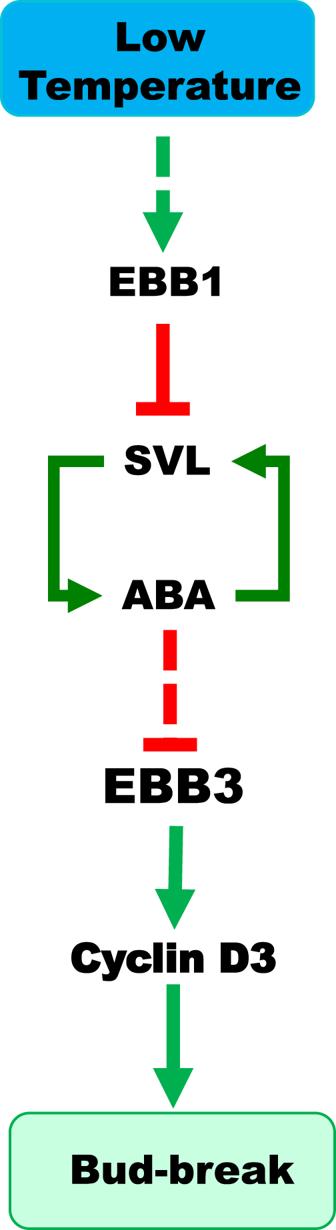Fig. 7: Hypothetical model of the roles EBB1, SVL and EBB3 play in control of bud-break in poplar. EBB1 is positively regulated by low temperature, leading to suppression ofSVLexpression. DecliningSVLexpression breaks the SVL/ABA feedforward loop. SVL/ABA repression leads to the upregulation ofEBB3and consequently to activation ofCYCD3.1, cell proliferation, and bud-break. Green arrows indicate positive regulation while red bars indicate negative regulation. Dash arrows indicate indirect regulation. See the text for additional description. Data were then filtered to remove adapters and trimmed for quality using Trimmomatic [60] (v0.36; settings TruSeq3-PE-2.fa:2:30:10 LEADING:3 SLIDINGWINDOW:5:20 MINLEN:50). After both filtering steps, FastQC was run again to ensure that no technical artefacts were introduced. Filtered reads were pseudo-aligned to v1.1 of the P. tremula transcripts [66] using kallisto [67] (v0.44; non default settings: -b 100 --rf-stranded -t 8). Statistical analysis of single-gene differential expression between conditions was performed in R [68] (v3.6.0) using the Bioconductor [69] (v3.9) DESeq2 package [70] (v1.20.1). FDR (False Discovery Rate) adjusted P -values were used to assess significance; a common threshold of 1% was used throughout. For the data quality assessment (QA) and visualisation, the read counts were normalised using a variance stabilising transformation as implemented in DESeq2. Reporting summary Further information on research design is available in the Nature Research Reporting Summary linked to this article.